Real-time observation of the charge transfer to solvent dynamics Intermolecular electron-transfer reactions have a crucial role in biology, solution chemistry and electrochemistry. The first step of such reactions is the expulsion of the electron to the solvent, whose mechanism is determined by the structure and dynamical response of the latter. Here we visualize the electron transfer to water using ultrafast fluorescence spectroscopy with polychromatic detection from the ultraviolet to the visible region, upon photo-excitation of the so-called charge transfer to solvent states of aqueous iodide. The initial emission is short lived (~60 fs) and it relaxes to a broad distribution of lower-energy charge transfer to solvent states upon rearrangement of the solvent cage. This distribution reflects the inhomogeneous character of the solvent cage around iodide. Electron ejection occurs from the relaxed charge transfer to solvent states with lifetimes of 100–400 fs that increase with decreasing emission energy. Outer-sphere electron-transfer reactions in water have been the subject of intense experimental and theoretical studies for decades, because of their importance in biology, solution chemistry and electrochemistry. The role of the solvent is crucial in affecting the outcome and efficiency of the reactions. The first step of an intermolecular electron-transfer reaction in solution is a charge transfer to solvent, which mediates the pathway between the donor and the acceptor. Several inorganic anions in polar solutions display characteristic broad ultraviolet absorption bands (peaking, for examples, for aqueous I − , at 225 and 193 nm) due to the charge-transfer-to-solvent (CTTS) states, which are quasi-bound states of the solute–solvent system with no equivalent for the isolated ions. The valence electrons of ground-state anions are bound by the nucleus, but the excited states are bound by solvent polarization [1] . The CTTS states of halides rapidly decay by ejection of an electron, which is then stabilized by solvation, leaving a neutral halogen atom behind [2] , [3] , [4] , [5] , [6] , [7] , [8] , [9] , [10] , [11] , [12] , [13] , [14] . Atomic anions are ideal for studies of the electron-transfer dynamics to the solvent, because the solute lacks internal (nuclear) degrees of freedom, such that the process of CTTS-mediated electron ejection is entirely governed by the structure and motions of the solvation shell. This also makes CTTS states ideal for probing the pure electronic solvation dynamics [15] . In a series of landmark papers, Sheu and Rossky [9] , [16] , [17] and Staib and Borgis [8] , [18] investigated by quantum simulations the dynamical evolution of the solvent ultimately leading to charge separation from the excited halide. Within the limits of their pioneering computational approach, they concluded that the detachment dramatically depends on the local water configuration around the ion, which should be reflected in a distribution of ejection times. More recently, Bradforth and Jungwirth [19] performed up-to-date computations of the electronic structure of the CTTS state of iodide in dynamical equilibrium with the water solvent. They concluded that the bulk wave function is mainly defined by the instantaneous location of voids in the first solvation shell, which arise due to thermal disorder in liquid water. Indeed, the shape and vertical excitation energy of the CTTS wave function of each excited ion were found to critically depend on the fluctuating local solvent arrangement. Finally, the key ingredient to CTTS binding in the bulk was found to be the long-range electrostatic field due to the pre-existing polarization of water molecules by the ground-state iodide ion [19] . Concerning the latter, molecular dynamics (MD) simulations with polarizable interaction potentials [20] showed that the solvent shell around (polarizable) iodide has an anisotropy that results from an induced dipole on the anion. This was later confirmed by quantum mechanics/molecular mechanics (QMMM) and full-quantum MD simulations [21] . These MD simulations show that overall, the protons of water point towards the iodide, but there is a large distribution of solvent cage configurations. From the experimental point of view, there has been a huge effort aimed at observing the early-time dynamics of aqueous CTTS states using ultrafast transient absorption (TA) spectroscopy [1] , [2] , [3] , [4] , [15] , [22] and, more recently, ultrafast photoemission from liquid microjets [5] , [6] . However, these methods turned out to be exclusively sensitive to the electron signal, that is, the end product of the photodetachment process, because of its very large oscillator strength over a broad spectral range and the fact that the excited CTTS absorption is close to that of the solvated electron [5] , [6] . These studies showed that in water the electron is detached from iodide in ~0.2 ps. Thereafter, relaxation of the host solvent cavity forms (in ~1 ps) a solvated electron [1] , [2] , [3] , [4] , [5] . Femtosecond X-ray absorption spectroscopy at the I L-edges detected the birth of the neutral halogen, but the time resolution was not sufficient to capture the early dynamics [7] . Of particular relevance here are the studies by Ruhman et al [11] , [12] and Schwartz et al [13] , [14] , [22] , [23] , [24] , [25] on the CTTS states of sodide (Na − ) in tetrahydrofuran (THF) and ether solvents, which enabled them to probe at high-time resolution both the signal of the ejected electron and the nascent neutral sodium atom. They found that electrons photodetached from the parent ion appear with their equilibrium spectrum after 500 fs with no further spectral evolution, nor a pump wavelength dependence. This led to the conclusion that electrons are ejected into pre-existing voids that are known to occur in room-temperature THF. Coming back to the case of the aqueous CTTS states, a direct way of probing their dynamics is by fluorescence at high temporal resolution. Indeed, CTTS transitions are strongly dipole-allowed (the integrated intensity of the first CTTS band yields a radiative lifetime of ~1 ns), therefore their fluorescence at early times, before complete electron-iodine separation, should be detectable. Indeed, with our fluorescence up-conversion setup, we detected short-lived emission (<50 fs) from molecular states with an order of magnitude longer radiative lifetimes [26] . Here, using the ultraviolet extension of our setup, we report the observation of the CTTS dynamics in real time. Upon excitation at the threshold of the CTTS absorption band (266 nm), which minimizes the excess energy in the system, of a 1 M aqueous iodide solution, we obtain the fluorescence spectrum shown in Fig. 1 . It consists of a very broad short-lived emission extending from the ultraviolet to the visible (VIS) region. The emission at λ <330 nm is very short lived, whereas for λ >330 nm, its lifetime increases with the wavelength, up to~400 fs. The extended energy range of the emission corresponds to excitation-emission Stokes shifts of ~0.3–~2.8 eV. To conclusively attribute this signal to the excitation of the iodide CTTS states, we verified that: (a) the emission intensity is linear with the iodide concentration from 200 mM to 6 M, with no changes in the dynamics ( Supplementary Fig. S1 ). This rules out higher-order processes, for example, recombination fluorescence between aqueous electrons and iodine; (b) the dynamics are independent of laser repetition rate ( Supplementary Fig. S2 ) excluding contributions from re-excited photoproducts; (c) the signal is linear with the pump intensity ( Supplementary Fig. S3 ), excluding multiphoton-excited emission from water or other species [27] ; (d) the dynamics are independent of the counter ion ( Supplementary Fig. S4 ); (e) we detected a comparable ultraviolet emission upon 255-nm excitation ( Supplementary Fig. S5 ); (f) similar results are obtained in D 2 O ( Supplementary Fig. S6 ). 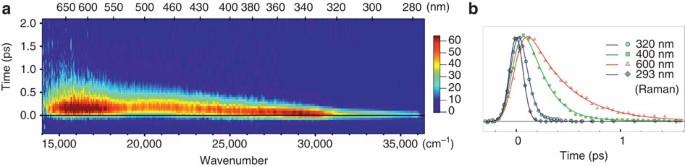Figure 1: Femtosecond fluorescence of aqueous iodine. (a) Fluorescence of 1 M NaI dissolved in water upon 266 nm excitation. The Raman signal from water was removed from the plot. (b) Normalized kinetic traces at different wavelengths with their representative fits (continuous lines), compared with the Raman signal from water at 293 nm, whose temporal width gives the IRF of the setup. Figure 1: Femtosecond fluorescence of aqueous iodine. ( a ) Fluorescence of 1 M NaI dissolved in water upon 266 nm excitation. The Raman signal from water was removed from the plot. ( b ) Normalized kinetic traces at different wavelengths with their representative fits (continuous lines), compared with the Raman signal from water at 293 nm, whose temporal width gives the IRF of the setup. Full size image A global analysis (see Methods) of the data gives the plots displayed in Fig. 2 . These show that the results are described by an ‘instantaneous’ excitation-emission Stokes shift of ~6,000 cm −1 , followed by dynamics with two time constants τ 1 =60±10 fs and < τ 2 >=250 fs. The former leads to the disappearance of the far ultraviolet side (>30,000 cm −1 ) of the emission, and to the concomitant growth, as a whole, of the emission between 15,000 and 30,000 cm −1 : this can be seen from the fact that the rise time is ~60 fs over the entire latter spectral region. The significant red shift (~10 4 cm −1 ) and broadening of the spectrum does not substantially change its total intensity, as seen by the lack of the 60 fs component in the kinetics of the integrated emission intensity ( Fig. 2b ). It is also worth noting that the short-lived far-ultraviolet emission is roughly the mirror image of the CTTS band, as expected immediately after excitation [26] . The second process ( τ 2 ) leads to the disappearance of the broad VIS signal. Its decay time increases from ~100 to ~400 fs, with increasing wavelength ( Fig. 2a ). Consistently with this distribution of rates, the overall intensity I decay ( Fig. 2b ) is well described by a stretched exponential function: log( I )~−( t / τ S ) γ , with τ S =210±20 fs and γ =0.79±0.05, which is a common phenomenological description of relaxation processes in disordered systems [28] . 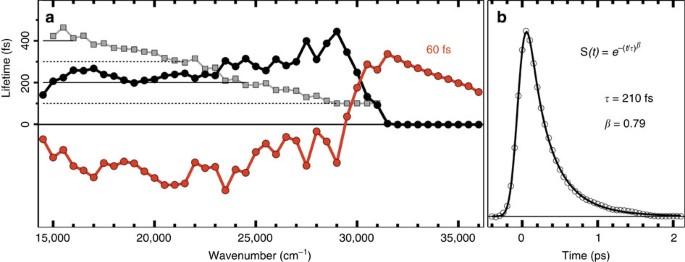Figure 2: Spectral decomposition analysis. (a) Global analysis of a comprehensive set of kinetic traces extracted fromFig. 1. The dynamics are described by two components: a fast component ofτ1=60 fs, whereas the longer one,τ2(λ), increases continuously with wavelength (grey squares). Red (black) dots are the amplitudes of the faster (slower) component. For the red curve, the positive part in the ultraviolet corresponds to a decay, whereas the negative portion in the VIS region (<30,000 cm−1) indicates a rise of the signal, both occurring with the sameτ1time constant. The black curve is the overall emission of the relaxed CTTS states (see text), which decay with multipleτ2time constants. (b) Kinetics of the intensity integrated over the entire spectral range (circles), fitted (black line) using a stretched exponential function convoluted with our IRF. Figure 2: Spectral decomposition analysis. ( a ) Global analysis of a comprehensive set of kinetic traces extracted from Fig. 1 . The dynamics are described by two components: a fast component of τ 1 =60 fs, whereas the longer one, τ 2 ( λ ), increases continuously with wavelength (grey squares). Red (black) dots are the amplitudes of the faster (slower) component. For the red curve, the positive part in the ultraviolet corresponds to a decay, whereas the negative portion in the VIS region (<30,000 cm −1 ) indicates a rise of the signal, both occurring with the same τ 1 time constant. The black curve is the overall emission of the relaxed CTTS states (see text), which decay with multiple τ 2 time constants. ( b ) Kinetics of the intensity integrated over the entire spectral range (circles), fitted (black line) using a stretched exponential function convoluted with our IRF. Full size image The value of < τ 2 > agrees with the ~0.2-ps appearance time of the TA signal of the aqueous electron [1] , [2] , [3] . Therefore, this process can safely be assigned to the conversion of the excited CTTS state to a non-emissive I 0 / e − pair, proceeding via charge transfer to water. However, two hitherto unreported [1] , [2] , [3] , [4] , [5] , [6] , [7] aspects of the aqueous CTTS dynamics are revealed here: (i) an early ( τ 1 ) relaxation of the CTTS with an upper limit of 60 fs, which leads to a distribution of relaxed excited electronic states from which actual ejection eventually occurs; these relaxed CTTS states are identified by their broad VIS emission ( Fig. 2 ); (ii) we find a wide range of τ 2 ejection rates that were not reported in the TA experiments on aqueous iodide [1] , [2] , [3] , [4] . This is not too surprising because the latter are only sensitive to the electron signal, and subsequent sub-picosecond solvent-relaxation processes around the electron [2] , [3] , [4] , [5] smear out the longer ejection times. On the other hand, because fluorescence occurs before complete electron-iodine separation, it avoids the latter effects and specifically visualizes the ejection event. The distribution of ejection times τ 2 ( λ ) reflects a variety of non-equivalent configurations of the relaxed CTTS state, due to the highly inhomogeneous character of the solvent shell and its anisotropy before excitation [19] , [20] , [21] , and to the fact that the shape of the CTTS wave function of each excited species critically depends on the local solvent arrangement, as stressed by Bradforth and Jungwirth [19] . As a consequence, we observe here that the initial water configurations around I − also determine the effective electron-departure timescales. For such a distribution of τ 2 times to arise, non-equivalent relaxed CTTS configurations must not interconvert within the decay time, because we observe the same rise of ~60 fs at all emission energies below ~30,000 cm −1 . Consistent with this are the characteristic response times of water, which contain a comparatively slower (~1 ps) component [29] , [30] , associated to collective long-range solvent rearrangements. Thus, it is the distribution of solvent shell configurations around I − that govern the electron-ejection rate. This is fully in line with Bradforth and Jungwirth [19] who stressed that the strong asymmetry of the environment predisposes the electron to bud in a defined direction. In this picture, the lower ejection rates correlate with solvent configurations of the CTTS that have relaxed to an energetically deeper minimum. The remarkable (>1 eV) energy dissipation shifting the emission from the ultraviolet to the VIS region in the first 60 fs is undoubtedly associated to close-range interactions with first-shell molecules readapting to the new charge distribution, as was already pointed out for I − in THF [24] . The 60-fs timescale points to an inertial (as opposed to diffusional) character of the solvent response [31] . Thereafter, there is still significant charge on iodine, or else the fluorescence would be strongly reduced by lack of radiative recombination of the electron and the hole. Simulations for chloride had suggested that within 100 fs after excitation a significant charge density still remains on Cl 0 , even if the centre of the electronic cloud has already shifted ~0.4 nm away [8] . The negligible (<10%) shortening of τ 1 from D 2 O to H 2 O ( Supplementary Fig. S6 ) indicates that the underlying solvent rearrangements are essentially translational, because for reorientation of water dipoles the timescale should scale as 2 1/2 by isotopic substitution [29] , [32] , [33] , [34] . As water reorientation is typically faster (10–30 fs (refs 29 , 30 , 31 , 32 , 33 , 34 )) than τ 1 =60 fs, it will adiabatically follow this translational rearrangement, the measured τ 1 representing a convolution of the two timescales. The simulations of Staib and Borgis [8] and Sheu and Rossky [9] predicted a large (>1 eV) and fast Stokes shift, which they attributed to the excited ion exerting forces that push the adjacent water molecules outwards. In this respect, because ground-state iodide is isoelectronic with xenon, one expects the excited CTTS state to resemble a diffuse, 6 s -like, Rydberg orbital (different from the much studied CTTS state of sodide, which has a p -like symmetry [10] ). Consistently, according to Bradforth and Jungwirth [19] , the CTTS wave function of iodide has the appearance of an orbital with a mixture of a major s -character and a smaller p -character, with a radial node similar to that of a hydrogenic 2 s wave function: on the whole, these properties are reminiscent of low- n Rydberg orbitals. In principle, this would imply an outward motion of the water molecules, due to the repulsion exerted by the excited orbital [35] , [36] . Furthermore, time-resolved X-ray absorption spectroscopy and MD simulations [7] showed that upon electron abstraction, the water molecules move outwards on the way to forming a hydrophobic solvation shell, because the interaction between water molecules is stronger than between water and iodine. However, the above two concurrent effects are idealized, and the process of electron ejection is complicated by the anisotropy of the solvent cage [20] , [21] and its dynamical character, which provides voids in the close vicinity of the anion into which the electron escapes. Indeed in Bradforth and Jungwirth [19] , it was found that the CTTS wave function has a minor lobe on iodine and a major one projecting the charge ~0.3 nm away into a void between the water molecules of its first solvation shell. These dynamically appearing voids are most likely related to the anisotropy of the solvent shell. At the other end of the reaction, the prevailing view of the solvated electron is that its s -like wave function resides in a nearly spherical cavity coordinated to 4–6 water molecules [37] , [38] , although recent work has shown that it may extend beyond the boundaries of this cavity [39] . The early time resemblance of the TA spectra [3] , [5] , [6] to that of the aqueous electron strongly suggests that at t ~0.2 ps, the structure of its first solvation shell of e − (H 2 O) is already very similar to the equilibrium one. The ejection distance upon excitation in the CTTS state at low energy was estimated to be ~0.5 nm [1] , [9] . Thus, the electron has to move ~0.2 nm through the initial solvent cage to go from the reactant to the product state. To make this possible, a major solvent rearrangement is needed: in particular, water molecules must move away in a non-isotropic fashion, either to clear the volume where the electron will eventually localize or where a void was present [8] , [9] , [19] . As the CTTS state and the ground state of the solvated electron have a similar, s -like symmetry, each CTTS state likely evolves on a single-potential energy surface all the way to the aqueous electron. This contrasts to the behaviour of, for example, Na − , whose CTTS state has a reversed, p -like symmetry such that a non-adiabatic transition is required to go from the reactant to the product state [13] . However, our findings show that the characteristic time scale of the dynamics (ultimately, the fluorescence lifetime) changes from excited ionic centre to the next because it strongly depends on the structure of the surrounding solvation cage at the time of photo-excitation. In summary, our experiments allow us to get a microscopic picture of the dynamics leading to electron detachment: after excitation, the closest water molecules quickly (~60 fs) readapt to the CTTS charge distribution by translating away. The external lobe of the CTTS wave function departs from iodide due to the anisotropy of the solvent cage and/or the occurrence of voids. In a way, there is some analogy with the mechanism reported for electron ejection in THF [12] , [22] , but the notion of pre-existing cavities in the latter is to be seen as of dynamical character in water. The solvent cage rearranges according to its initial structure, giving rise to the relaxed CTTS state. In this step, energy dissipation has strongly shifted the fluorescence, but its intensity is undiminished, because radiative emission mainly arises from the residual electronic density in the internal lobe localized on I 0 , which overlaps with the ground-state wave function. Ejection of the electron into the solvent consists in the complete disappearance of this residual charge on the ion, which irreversibly quenches the fluorescence. As argued above, this final step is driven by diffusional (~0.25–1 ps) rearrangement of H 2 O molecules belonging to several solvation shells around iodine. Experimental setup Time-resolved emission measurements were carried out by the fluorescence up-conversion technique in the ultraviolet region [40] . Briefly, a Coherent-RegA Ti:Sapphire regenerative amplifier provided 800 nm pulses of 4 μJ typical energy and 80 fs duration (full width at half maximum (FWHM) of the intensity autocorrelation curve). The amplified laser system was operated at 150 kHz, except for the measurement at 15 kHz shown in Supplementary Fig. S2 . About 1/3 of this beam was tripled to yield excitation pulses at 266 nm, 40 nJ per pulse typical energy. The excitation beam was focused down to a 30-μm spot inside a 0.2-mm thick ultraviolet-grade glass flow cell where the sample was continuously circulated at room temperature at a typical speed of 1 m s −1 . In these conditions, the excitation pulses hit the same spot ~8 times. Emission from the sample was collected by a parabolic mirror in forward-scattering geometry, and directed to a second mirror that focused it to a β-barium borate (BBO) crystal. The emission was then up-converted at the focal point by mixing it in a slightly non-collinear geometry with a gate pulse at 800 nm obtained from the residual portion of the fundamental beam. The intensity of the gate beam was properly adjusted to eliminate the background signal due to harmonic generation inside the up-conversion BBO. The up-converted signal was spatially filtered and detected with a spectrograph and a liquid-N 2 -cooled CCD (charge-coupled device) camera. Kinetic traces at a fixed wavelength were obtained by scanning the delay stage while keeping the BBO crystal at a given angle. Polychromatic detection was obtained by rotating the BBO crystal by a computer-controlled motor during the accumulation time of the CCD camera to phase match a wide spectral region at each time delay. Because of the very wide spectral extension of the signal, we measured independently the ultraviolet (270–400 nm) and VIS (400–750 nm) emission regions by using two different BBO crystals (of 0.10 and 0.25 mm thicknesses, respectively) and then joined the two measurements to obtain the overall spectrum. For the VIS measurement, an appropriate Schott filter was used to attenuate the residual excitation beam. Each measurement reported here is the average of ~30 scans. This corresponds to an integration time on the CCD of ~2 h to acquire the complete spectrum at each delay time. No significant variations were observed from scan to scan, and the laser intensity was verified before and after each measurement. The acquired spectra were corrected by the spectral response of the setup, estimated by comparing the time-integrated emission of several known dyes with their static spectra known from literature. All measurements were carried out at room temperature. The Raman signal between 290 and 296 nm was removed from Fig. 1a via a linear interpolation procedure. We estimated a ~150-fs Gaussian instrumental response function (IRF) of the setup by measuring the FWHM of a kinetic trace of the Raman line of H 2 O excited at 266 nm. This value might become slightly longer in the VIS because we used a thicker BBO crystal. We estimated an upper limit of 170 fs by observing the rise time of the signal in a known dye. Given the typical signal/noise ratio of our measurements, these values of the IRF lead to a value of ~40 fs as the shortest (exponential) decay time we are able to detect reliably (compare, for example, in Fig. 1b the Raman trace with the signal at 320 nm). Samples Samples consisted of aqueous solutions of NaI and KI at different concentrations. We used a concentration of 1 M to measure the signal in Fig. 1 . This corresponds to ~0.18 optical density absorption through the flow cell at the 266-nm excitation wavelength. Static absorption measurements were carried out on a Shimadzu UV-3600 spectrophotometer. No significant variations of the absorption spectrum were observed after each experiment. NaI and KI of purity ranging from 99 to 99.999% were obtained by Fluka, Aldrich and Alfa Aesar. The samples were prepared by using deionized water, high-purity distilled water obtained by Gibco and high-purity D 2 O obtained by Aldrich. We found no dependence of any of the observed dynamics on the purity level of both the solute and the solvent. Data analysis The global analysis in Fig. 2 was carried out by least-square fitting simultaneously a set of 44 representative kinetic traces obtained by cuts of data in Fig. 1 at different wavelengths. We used the following fitting function: where IRF( t ) represents our Gaussian IRF of 150 fs FWHM, the dot indicates convolution over time, and τ 1 , A 1 ( λ ), τ 2 ( λ ), and A 2 ( λ ) are the free parameters of the fit. This expression represents two dynamics (no. 1 and 2) with characteristic timescales τ 1 and τ 2 ( λ ). Although the former was assumed to be constant throughout the spectrum, a continuous wavelength dependence of the timescale of process no. 2 was needed to reproduce the data. A 1 ( λ ) and A 2 ( λ ) are the decay-associated spectra (DAS) of process no. 1 and 2, respectively, shown as red and black curves in Fig. 2 , respectively. Based on expression (1), a positive value of A ( λ ) corresponds to a decay, whereas a negative value implies a rise. Hence (see Fig. 2 ), the DAS of process 1 represents a decay in the ultraviolet portion of the signal accompanied by a rise of the emission in the VIS region. The DAS of process 2 is positive throughout the spectrum and thus it represents a decaying signal. It is worth noting that theory predicts the shortest (sub-100 fs) solvation-induced relaxation we observed in this work to be a Gaussian kinetics, exp[− t 2 /(2 τ G 2 )], rather than by an exponential one [18] , [29] , [30] , [31] , [33] , [41] . This is because of the fact that the ultrafast component of solvent relaxation is mainly driven by the inertial, non-diffusive response of water molecules. However, although we are able to estimate by deconvolution the timescale of a process as fast as ~40 fs, our technique is not sufficiently sensitive to the detailed shape of an ultrafast (sub-IRF) decay. As a matter of fact, we cannot reliably distinguish between a Gaussian and an exponential form of such a fast decay kinetics, both evenly fitting the observed kinetics ( Supplementary Fig. S7 ). For these reasons and for the sake of simplicity, we used an exponential fit, rather than a Gaussian one. This procedure has already been used in previous works [31] , [41] and does not affect the estimate of the characteristic timescale of the processes, which is the main aim of our analysis. The overall intensity of the signal in Fig. 2b was obtained by numerical integration of the data on the whole spectral range. This kinetics was fitted by a stretched exponential function, log I ~−( t / τ S ) γ , convoluted with our Gaussian IRF. Although the stretched exponential has only a phenomenological meaning, from the best-fit parameters, τ S =210±20 fs and γ =0.79±0.05, one can estimate [28] the average and s.d. of the underlying distribution of decay times to be 240 and 135 fs, respectively. These values are consistent with the observed dispersion of τ 2 (grey points in Fig. 2a ) from 100 to 450 fs around an average of < τ 2 >=250 fs. How to cite this article: Messina, F. et al. Real-time observation of the charge transfer to solvent dynamics. Nat. Commun. 4:2119 doi: 10.1038/ncomms3119 (2013).